Mitochondrial respiration protects against oxygen-associated DNA damage Oxygen is not only required for oxidative phosphorylation but also serves as the essential substrate for the formation of reactive oxygen species (ROS), which is implicated in ageing and tumorigenesis. Although the mitochondrion is known for its bioenergetic function, the symbiotic theory originally proposed that it provided protection against the toxicity of increasing oxygen in the primordial atmosphere. Using human cells lacking Synthesis of Cytochrome c Oxidase 2 ( SCO2−/− ), we have tested the oxygen toxicity hypothesis. These cells are oxidative phosphorylation defective and glycolysis dependent; they exhibit increased viability under hypoxia and feature an inverted growth response to oxygen compared with wild-type cells. SCO2−/− cells have increased intracellular oxygen and nicotinamide adenine dinucleotide (NADH) levels, which result in increased ROS and oxidative DNA damage. Using this isogenic cell line, we have revealed the genotoxicity of ambient oxygen. Our study highlights the importance of mitochondrial respiration both for bioenergetic benefits and for maintaining genomic stability in an oxygen-rich environment. The earth has been anaerobic and hypoxic for much of its 4.5 billion-year history. The relatively late rise in ambient oxygen likely required organisms to evolutionarily adapt to life in an oxygen-rich, oxidative environment [1] . The symbiotic theory of the origin of the modern-day mitochondrion holds that the engulfment of aerobic proteobacteria by primordial anaerobic eukaryotes may have provided protection against oxygen toxicity [2] . Although the mitochondrion has been extensively studied from the perspective of energy homeostasis, the originally proposed protective role against oxygen toxicity has received less attention. Recent studies suggest that improving mitochondrial function reduces the deleterious effects of oxidative stress such as ageing, cancer, metabolic and neurodegenerative diseases [3] , [4] , [5] , [6] , [7] . The concordance of these observations across species from yeast to mammal indicates that other effects of mitochondrial respiration beyond bioenergetic function may be important for aerobic life. Tumorigenesis is thought to be driven by the multistep acquisition of mutations caused by genotoxic stresses, such as DNA damaging agents and reactive oxygen species (ROS). Among the many transcriptional targets of the tumour suppressor gene p53 are antioxidant enzymes and the RRM2B gene encoding the regulatory subunit of ribonucleotide reductase, which prevents mitochondrial DNA depletion and dysfunction [8] , [9] , [10] . The tumour suppressor encoded by the ATM gene, a critical mediator of DNA damage responses, has also been shown to stabilize mitochondrial DNA through regulation of ribonucleotide reductases in a tissue-specific manner [11] . These observations implicate ROS in tumorigenesis and suggest that the optimization of mitochondrial function, possibly through redox and maintenance of intracellular oxygen homeostasis, has a protective role against oxidative damage to genomic DNA. In bacteria, physiological levels of oxygen have been shown to be mutagenic [12] . Whether the reduction of oxygen by respiration in human cells protects against DNA damage-induced growth arrest or tumour-promoting mutations remains to be genetically demonstrated. Although many studies have linked oxidative stress and cancer, clinical investigations have not uniformly demonstrated a benefit of antioxidants against cancer, and the use of these drugs as chemopreventives remains controversial [13] , [14] , [15] , [16] . Such disparate observations indicate a need to better understand the cellular control of oxygen use and the relationship between oxidative stress and tumorigenesis. We recently reported the regulation of mitochondrial respiration by p53 through its transcriptional target gene Synthesis of Cytochrome c Oxidase 2 ( SCO2 ) [17] . The SCO2 protein is essential for the assembly of the mitochondrial cytochrome c oxidase (COX) complex (IV), the metabolic centre of eukaryotic oxygen consumption [18] , [19] . Although the biological significance of the p53/SCO2 pathway remains to be clarified, the major role of p53 as 'guardian of the genome' [20] , [21] would suggest that the regulation of respiration may confer genomic protection. We tested this hypothesis by genetically disrupting SCO2 , thereby eliminating mitochondrial respiration, in a human cell line. Indeed, loss of respiration disrupts redox homeostasis and increases the intracellular oxygen availability that contributes to increased ROS formation and oxidative DNA damage. Thus, our genetic study demonstrates the importance of optimizing mitochondrial function, which when dysfunctional has been proposed to lie at the core of degenerative diseases related to ageing and cancer [22] . Eliminating oxidative phosphorylation reveals oxygen toxicity To create a stable, respiration-deficient cell line isogenically matched to respiration-competent cells, we sequentially disrupted both alleles of the SCO2 gene in the human colon cancer cell line HCT116 by homologous recombination [23] , [24] . HCT116 cells have wild-type p53 alleles and can robustly upregulate SCO2 expression in response to DNA damage [25] . Targeting vectors were delivered by recombinant adeno-associated virus; a PCR screen was used to isolate homologous recombinants [17] , [24] , [26] . The disruption of both SCO2 alleles was confirmed by the complete absence of SCO2 protein expression ( Fig. 1a ). SCO2−/− cells exhibited a marked reduction in oxygen consumption compared with parental cells ( SCO2+/+ ), indicating a cessation of oxidative phosphorylation and a compensatory increase in lactate production ( Fig. 1a ). A greater dependence on glucose for growth of SCO2−/− cells indicated a switch in metabolism to glycolysis for adenosine triphosphate (ATP) generation ( Fig. 1b ). It is notable that the magnitude of increase in lactate generation did not seem sufficient to compensate for the loss of oxidative phosphorylation in SCO2−/− cells. Other than insufficient energy generation by glycolysis, impaired glutaminolysis, which also generates lactate and supports anabolic requirements, may be another contributing factor to the approximately twofold longer doubling time ( ∼ 48 h) of SCO2−/− cells [27] . 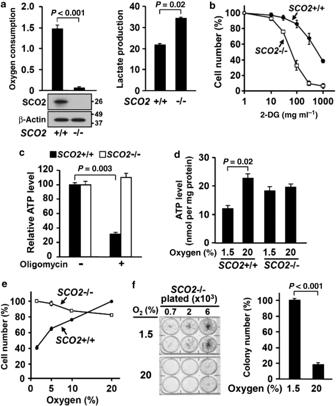Figure 1: Disruption of respiration dissociates the toxic effects of oxygen from the bioenergetic benefits of oxidative phosphorylation. Recombinant adeno-associated virus-mediated homologous recombination was used to derive human HCT116 cell lines with biallelically disruptedSCO2(SCO2−/−)24. (a) SCO2 protein assessed by western blotting. β-Actin was probed as loading control. Whole-cell oxygen consumption measurements in nmol per min per 106cells and lactate generation in nmol per min per mg protein (n=3). (b) Growth sensitivity ofSCO2+/+andSCO2−/−cells to 2-deoxy-D-glucose (2-DG) (n=3). (c) The relative total cellular ATP levels ofSCO2+/+ andSCO2−/−cells before and after oligomycin addition are shown (n=3). (d) Effect of ambient oxygen on steady-state ATP levels, in nmol per mg protein (n=4). (e) Relationship between oxygen and cell growth in non-respiring (SCO2−/−) cells compared with respiring (SCO2+/+) cells. The cell number at each oxygen concentration is represented as a percentage of the optimal oxygen concentration, 20% oxygen forSCO2+/+and 1.5% oxygen forSCO2−/−cells. Average values are from three independent experiments performed in duplicate (n=3). (f) Rescue ofSCO2−/−cell-colony formation by hypoxia (1.5% oxygen). Representative colony formation assay plates are shown forSCO2−/−cells plated at different densities, which were quantified by counting colony number (n=4). Values are shown as mean and s.e.m.;P-values determined by Student'st-test. Figure 1: Disruption of respiration dissociates the toxic effects of oxygen from the bioenergetic benefits of oxidative phosphorylation. Recombinant adeno-associated virus-mediated homologous recombination was used to derive human HCT116 cell lines with biallelically disrupted SCO2 ( SCO2−/− ) [24] . ( a ) SCO2 protein assessed by western blotting. β-Actin was probed as loading control. Whole-cell oxygen consumption measurements in nmol per min per 10 6 cells and lactate generation in nmol per min per mg protein ( n =3). ( b ) Growth sensitivity of SCO2+/+ and SCO2−/− cells to 2-deoxy- D -glucose (2-DG) ( n =3). ( c ) The relative total cellular ATP levels of SCO2 +/+ and SCO2−/− cells before and after oligomycin addition are shown ( n =3). ( d ) Effect of ambient oxygen on steady-state ATP levels, in nmol per mg protein ( n =4). ( e ) Relationship between oxygen and cell growth in non-respiring ( SCO2−/− ) cells compared with respiring ( SCO2+/+ ) cells. The cell number at each oxygen concentration is represented as a percentage of the optimal oxygen concentration, 20% oxygen for SCO2+/+ and 1.5% oxygen for SCO2−/− cells. Average values are from three independent experiments performed in duplicate ( n =3). ( f ) Rescue of SCO2−/− cell-colony formation by hypoxia (1.5% oxygen). Representative colony formation assay plates are shown for SCO2−/− cells plated at different densities, which were quantified by counting colony number ( n =4). Values are shown as mean and s.e.m. ; P -values determined by Student's t -test. Full size image Non-respiring SCO2−/− cells would be predicted to be oxygen independent for energy generation because they do not carry out oxidative phosphorylation, as confirmed by unchanged ATP levels after oligomycin addition ( Fig. 1c ). Although the steady-state ATP levels in SCO2−/− cells were not significantly different compared with wild-type cells in 20% oxygen (room air), there was a markedly differential response to oxygen. The ATP level in SCO2−/− cells was unaltered by lower oxygen concentrations in contrast to the decrease in SCO2+/+ cells ( Fig. 1d ). When we compared growth in the range of 1.5–20% ambient oxygen, the relationship between cell proliferation and oxygen was essentially reversed in non-respiring cells compared with respiring cells, that is, growth of SCO2+/+ cells was stimulated by increasing oxygen levels, whereas growth of SCO2−/− cells was suppressed ( Fig. 1e ). To confirm the growth inhibitory effect of oxygen on non-respiring cells, we examined the effect of oxygen on the survival of SCO2+/− cells after integration of the SCO2 targeting vector. This experiment simultaneously generated homozygous knockout clones, in which the remaining wild-type SCO2 allele in cells was disrupted by homologous integration, and heterozygous clones in which the targeting vector had integrated randomly. In 20% oxygen, the fraction of PCR-positive SCO2−/− clones recovered was 0.3% (3 out of 892 total transgenic clones) compared with 4% (4 out of 96 transgenic clones) grown under the 1.5% oxygen selection condition (Fisher's exact test, P <0.003). The more than 10-fold higher efficiency of SCO2−/− clonal growth under hypoxic conditions indicated that ambient air may be toxic to non-respiring cells. The increased sensitivity of SCO2−/− cells to oxygen was further demonstrated by the dramatic rescue of colony formation under 1.5 versus 20% oxygen condition ( Fig. 1f ). Subsequent to these observations, expanded clones of SCO2−/− cells were maintained in the 1.5–5% oxygen range for optimal growth before experimental manipulations. Because differences in adaptation after loss of respiration may result in variable clonal phenotypes, we confirmed our results with an independently derived SCO2−/− cell line ( Supplementary Fig. 1 ). Altered redox and oxygen homeostasis underlie oxygen toxicity SCO2+/+ cells demonstrated bioenergetic dependence on oxidative phosphorylation as evidenced by a positive relationship between ATP levels and oxygen ( Fig. 1d ). In contrast, SCO2−/− cell growth was inhibited by increasing oxygen concentrations without associated changes in ATP levels ( Fig. 1d,e ). These results suggested that the sensitivity of SCO2−/− cells to oxygen was independent of cellular energy requirements and was instead caused by oxygen toxicity through the generation of ROS. To explore this possibility, we measured intracellular ROS levels by using the hydrogen peroxide-sensitive dye dichlorofluorescein (DCF). In comparison with their wild-type counterparts, SCO2−/− cells had markedly elevated levels of ROS as indicated by DCF staining intensity ( Fig. 2a ). This was reversed by the addition of the antioxidant N -acetyl- L -cysteine (NAC). To determine whether increased ROS was associated with the growth inhibition of SCO2−/− cells by oxygen, colony formation was examined in the presence of NAC, which essentially reversed the inhibitory effect of 20% oxygen on cell growth, implicating ROS as an aetiological agent ( Fig. 2b ). 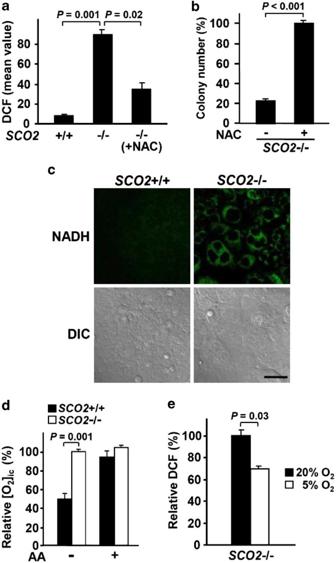Figure 2: Disruption of respiration increases ROS levels in association with increased reducing equivalents and intracellular oxygen. (a) Relative ROS levels in the respective cells types quantified by DCF FACS of whole cells.SCO2−/−cells were treated with NAC for 24 h before ROS measurement (n=3). (b) Rescue ofSCO2−/−cell-colony formation by 3 mM NAC in 20% oxygen condition. Colony formation ofSCO2−/−cells with or without NAC was quantified (n=4). (c) Cellular NADH levels in attachedSCO2+/+andSCO2−/−cells imaged by ultraviolet laser confocal microscopy (green fluorescence). Differential interference contrast (DIC) phase images show the respective cell densities. Scale bar, 50 μm. (d) Relative intracellular oxygen levels ([O2]ic) were quantified using high-resolution fluorescent microscopy after transfection of the phosphorescent oxygen-sensitive probe IC60N. Measurements were performed in a 5% ambient oxygen-controlled chamber. Complex III inhibitor antimycin A (+AA, 5 μM) was added to demonstrate the dependence of [O2]icon active respiration. The [O2]iclevels shown are relative to those in non-respiringSCO2−/−cells in 5% oxygen-saturated medium (n=7). (e) Effect of ambient oxygen on ROS production inSCO2−/−cells. Cells were maintained at the indicated oxygen concentration for 7–10 days before DCF FACS analysis (n=3). Values shown as mean and s.e.m.;P-values determined by Student'st-test. Figure 2: Disruption of respiration increases ROS levels in association with increased reducing equivalents and intracellular oxygen. ( a ) Relative ROS levels in the respective cells types quantified by DCF FACS of whole cells. SCO2−/− cells were treated with NAC for 24 h before ROS measurement ( n =3). ( b ) Rescue of SCO2−/− cell-colony formation by 3 mM NAC in 20% oxygen condition. Colony formation of SCO2−/− cells with or without NAC was quantified ( n =4). ( c ) Cellular NADH levels in attached SCO2+/+ and SCO2−/− cells imaged by ultraviolet laser confocal microscopy (green fluorescence). Differential interference contrast (DIC) phase images show the respective cell densities. Scale bar, 50 μm. ( d ) Relative intracellular oxygen levels ([O 2 ] ic ) were quantified using high-resolution fluorescent microscopy after transfection of the phosphorescent oxygen-sensitive probe IC60N. Measurements were performed in a 5% ambient oxygen-controlled chamber. Complex III inhibitor antimycin A (+AA, 5 μM) was added to demonstrate the dependence of [O 2 ] ic on active respiration. The [O 2 ] ic levels shown are relative to those in non-respiring SCO2−/− cells in 5% oxygen-saturated medium ( n =7). ( e ) Effect of ambient oxygen on ROS production in SCO2−/− cells. Cells were maintained at the indicated oxygen concentration for 7–10 days before DCF FACS analysis ( n =3). Values shown as mean and s.e.m. ; P -values determined by Student's t -test. Full size image SCO2−/− cells also displayed high levels of nicotinamide adenine dinucleotide (NADH) because of the disruption of electron flow to molecular oxygen ( Fig. 2c ). We speculated that in the absence of its consumption, intracellular oxygen levels may be increased and may more readily contribute to increased ROS formation in such a highly reduced, electron-rich environment. We used a recently developed oxygen-sensitive probe to measure intracellular oxygen concentration ([O 2 ] ic ) under near-physiological tissue oxygen conditions ( ∼ 5%) to more closely mimic the effect of respiration on intracellular oxygen homeostasis [28] , [29] , [30] . As predicted, the intracellular oxygen concentration in non-respiring SCO2−/− cells was higher than in SCO2+/+ cells ( Fig. 2d ). This relative oxygen gradient required respiration, as demonstrated by the addition of complex III inhibitor antimycin A, which eliminated the difference between SCO2+/+ and SCO2−/− cells. Decreasing ambient oxygen exposure of SCO2−/− cells significantly reduced ROS levels, providing further support for a mechanistic link between intracellular oxygen availability and ROS generation in mitochondrial dysfunction ( Fig. 2e ). These cell-based findings are consistent with recent results from an in vivo ageing model [7] that suggests that active mitochondrial respiration can impact the homeostasis of intracellular oxygen involved in ROS formation. Furthermore, recent studies have shown that mitochondrial ROS production is significantly dependent on oxygen levels that are generally lower under physiological conditions compared with in vitro experiments performed under room air [28] , [30] , [31] , [32] . What is the source of increased ROS in SCO2−/− cells? ROS are generated by mitochondria and by cytoplasmic oxidoreductases. The basal ROS level in SCO2−/− cells was significantly attenuated by the cytoplasmic NADPH oxidoreductase blocker diphenyliodonium, as compared with parental cells, whereas electron transport chain inhibitors had no differential effect ( Supplementary Fig. 2a ). Purified mitochondria from SCO2−/− cells exhibited no difference in basal ROS production when compared with those derived from wild-type cells and showed no increase when treated with respiratory inhibitors. These results are consistent with the absence of electron transport in SCO2−/− cells and support a cytoplasmic source of ROS ( Supplementary Fig. 2b ). Ambient oxygen contributes to oxidative DNA damage An important consequence of increased oxidative stress is genomic DNA damage. If increased intracellular oxygen availability is indeed important for ROS generation, modulating ROS by altering ambient oxygen in non-respiring cells should directly affect oxidative DNA damage. We examined DNA damage under different ambient oxygen concentrations by measuring modified DNA base 8-oxoguanine (8-oxoG) immunofluorescence. SCO2−/− cells exhibited relatively higher 8-oxoG levels with increasing ambient oxygen, compared with SCO2+/+ cells ( Fig. 3a ). The observation of higher oxygen-dependent DNA damage in SCO2−/− cells was also suggested by increases in the levels of DNA damage response phosphoprotein γ-H2AX observed by western blotting ( Fig. 3b ). There were parallel increases in p53 protein, another sensitive marker of DNA damage ( Fig. 3b ). Despite evidence of DNA damage response in SCO2−/− cells, neither apoptosis nor necrosis was increased compared with SCO2+/+ cells at baseline ( Supplementary Fig. 3 ) [24] . This suggests the presence of effective adaptive mechanisms for the survival of cells with mitochondrial dysfunction, such as through Polo-like kinases 1 and 2, which seem to be essential for their viability [24] . However, Polo-like kinase 2 expression was not increased by hypoxia in SCO2−/− cells, further supporting decreased DNA damage associated with reduced ambient oxygen as being the major contributing factor for their improved colony formation ( Fig. 1f , Supplementary Fig. 4 ). 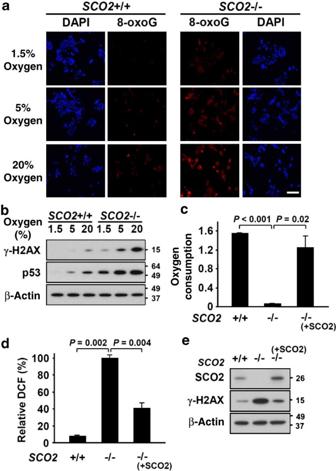Figure 3: Effect of ambient oxygen on the inverse relationship between respiration and oxidative DNA damage and DNA damage response. (a) Visualization of oxidized DNA marker 8-oxoguanine (8-oxoG) by immunofluorescence (secondary antibody labelled with Alexa red) in respiring (SCO2+/+) versus non-respiring (SCO2−/−) cells incubated in 1.5%, 5 or 20% oxygen condition. Nuclei are counterstained with 4,6-diamidino-2-phenylindole (DAPI) (blue). Scale bar, 50 μm. (b) Relative quantification of two DNA damage response proteins, γ-H2AX and p53, by western blotting in response to increasing ambient oxygen. All cells were incubated for 48 h in the indicated oxygen condition before analysis. Lentivirus-mediated re-introduction of exogenous SCO2 intoSCO2−/−cells: (c) rescues respiration; (d) reverses the increase in ROS; and (e) reduces DNA damage response (n=3). Values are shown as mean and s.e.m.;P-values determined by Student'st-test. Figure 3: Effect of ambient oxygen on the inverse relationship between respiration and oxidative DNA damage and DNA damage response. ( a ) Visualization of oxidized DNA marker 8-oxoguanine (8-oxoG) by immunofluorescence (secondary antibody labelled with Alexa red) in respiring ( SCO2+/+ ) versus non-respiring ( SCO2−/− ) cells incubated in 1.5%, 5 or 20% oxygen condition. Nuclei are counterstained with 4,6-diamidino-2-phenylindole (DAPI) (blue). Scale bar, 50 μm. ( b ) Relative quantification of two DNA damage response proteins, γ-H2AX and p53, by western blotting in response to increasing ambient oxygen. All cells were incubated for 48 h in the indicated oxygen condition before analysis. Lentivirus-mediated re-introduction of exogenous SCO2 into SCO2−/− cells: ( c ) rescues respiration; ( d ) reverses the increase in ROS; and ( e ) reduces DNA damage response ( n =3). Values are shown as mean and s.e.m. ; P -values determined by Student's t -test. Full size image Respiration protects against oxygen-associated DNA damage To confirm that disruption of respiration caused DNA damage in SCO2−/− cells, we first stably re-expressed SCO2 protein and thereby rescued their respiratory capacity ( Fig. 3c ). There was a tight concordance between increased respiration and decreased ROS and DNA damage response ( Fig. 3c–e ). 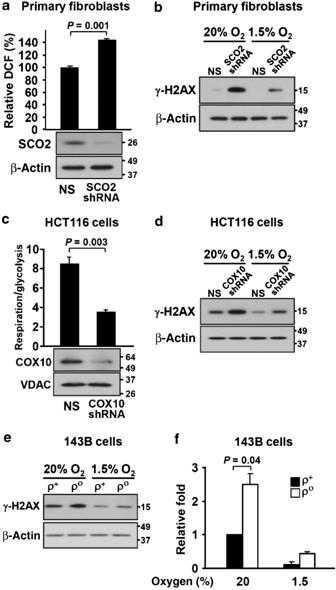Figure 4: Disruption of respiration increases ROS and DNA damage response in both primary human fibroblasts and other cancer cells. (a) Human fibroblasts were stably transduced with nonspecific (NS) or SCO2 short hairpin RNA (shRNA) and ROS levels were analysed by FACS (n=3). Western blotting was conducted to confirm SCO2 knockdown. β-Actin serves as loading control. (b) Effect of SCO2 knockdown on γ-H2AX in primary fibroblasts and its sensitivity to ambient oxygen. (c) The COX10 subunit was knocked down in HCT116SCO2+/+ cells by stable shRNA transduction and was confirmed by western blotting versus nonspecific (NS) shRNA. VDAC serves as loading control. Functional disruption of respiration was confirmed by oxygen consumption and extracellular acidification ratios (respiration/glycolysis) using a Seahorse Bioscience XF24 instrument (n=5). (d) Effect of COX10 knockdown on γ-H2AX in HCT116SCO2+/+ cells and its sensitivity to ambient oxygen. (e) DNA damage response in non-respiring human osteosarcoma 143B ρocells versus respiring 143B ρ+cells and its sensitivity to ambient oxygen. β-Actin serves as protein loading control. (f) Quantification of the DNA damage response by densitometric scanning of γ-H2AX protein levels normalized by β-actin in 143B cells (n=3). Values shown as mean and s.e.m.;P-values are determined by Student'st-test. To ensure these findings were not limited to the HCT116 cell line, we knocked down SCO2 using short hairpin RNA in primary human fibroblasts and observed similar increases in DNA damage responses that were sensitive to ambient oxygen and increased ROS levels ( Fig 4a,b ). To rule out the possibility that functions of SCO2 unrelated to respiration might contribute to the DNA damage response observed, we generated a stable cell line expressing short hairpin RNA targeted against COX10, another assembly protein of the COX complex, the absence of which disrupts respiration [33] . Similar to the genetic disruption of SCO2, the depletion of COX10 protein resulted in decreased respiration and a DNA damage response that was sensitive to ambient oxygen levels ( Fig. 4c,d ). As an additional control, we tested mtDNA-depleted rho zero (ρ o ) cells matched to control (ρ + ) cells, another model of mitochondrial dysfunction in a different cell line, and observed a similar relationship between oxygen and DNA damage response as seen in SCO2−/− HCT116 cells ( Fig. 4e,f ). Figure 4: Disruption of respiration increases ROS and DNA damage response in both primary human fibroblasts and other cancer cells. ( a ) Human fibroblasts were stably transduced with nonspecific (NS) or SCO2 short hairpin RNA (shRNA) and ROS levels were analysed by FACS ( n =3). Western blotting was conducted to confirm SCO2 knockdown. β-Actin serves as loading control. ( b ) Effect of SCO2 knockdown on γ-H2AX in primary fibroblasts and its sensitivity to ambient oxygen. ( c ) The COX10 subunit was knocked down in HCT116 SCO2 +/+ cells by stable shRNA transduction and was confirmed by western blotting versus nonspecific (NS) shRNA. VDAC serves as loading control. Functional disruption of respiration was confirmed by oxygen consumption and extracellular acidification ratios (respiration/glycolysis) using a Seahorse Bioscience XF24 instrument ( n =5). ( d ) Effect of COX10 knockdown on γ-H2AX in HCT116 SCO2 +/+ cells and its sensitivity to ambient oxygen. ( e ) DNA damage response in non-respiring human osteosarcoma 143B ρ o cells versus respiring 143B ρ + cells and its sensitivity to ambient oxygen. β-Actin serves as protein loading control. ( f ) Quantification of the DNA damage response by densitometric scanning of γ-H2AX protein levels normalized by β-actin in 143B cells ( n =3). Values shown as mean and s.e.m. ; P -values are determined by Student's t -test. Full size image The association between mitochondrial respiration and DNA damage response in non-genetically altered human cells was examined using chemical inhibitors against three mitochondrial respiratory complexes. The acute pharmacological disruption of electron transfer in SCO2+/+ cells resulted in increased γ-H2AX levels in 20% oxygen ( Fig. 5a ). However, no effect of these agents was observed in SCO2−/− cells, which also exhibited unchanged levels of ROS in response to these agents ( Fig. 5a , Supplementary Fig. 2 ). Importantly, the relative difference in the DNA damage response between SCO2+/+ and SCO2−/− cells after treatment with respiratory inhibitors could be attenuated by decreasing ambient oxygen, reflecting the contribution of intracellular oxygen to oxidative DNA damage ( Fig. 5a ). 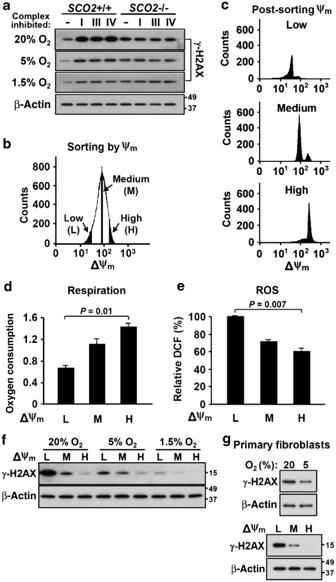Figure 5: Respiration is inversely related to DNA damage response in genetically unmodified cancer cells and primary fibroblasts. (a) Respiration in HCT116SCO2+/+cells was inhibited by acutely targeting each of the three respiratory complexes with the indicated agents for 24 h (I=rotenone, 0.1 μM; III=antimycin A, 3 mM; IV=potassium cyanide, 0.1 mM). DNA damage responses under indicated ambient oxygen conditions were monitored by γ-H2AX western blotting. As negative control, note the lack of DNA damage response in non-respiringSCO2−/−cells. (b)SCO2+/+cells maintained under indicated oxygen conditions were FACS sorted by mitochondrial membrane potential using potentiometric dye JC-1 and divided into a low (L), medium (M) or high (H) mitochondrial membrane potential sub-population (∼5 to 10% of the total population). The viability of all three fractions was greater than 96–99% by Trypan blue dye exclusion. (c) The stability of the mitochondrial membrane potential of postsorted cells was confirmed by FACS at the same setting. (d) Whole-cell oxygen consumption measurements in L, M and H mitochondrial membrane potential sub-populations (nmol per min per 106cells) (n=3). (e) Relative ROS levels in the respective fractions quantified by DCF FACS (n=3). (f) Relative DNA damage response in the respective fractions determined by γ-H2AX western blotting. (g) DNA damage response of primary mouse embryo fibroblasts under the indicated ambient oxygen conditions, as well as after FACS sorting into L, M and H mitochondrial membrane potential sub-populations in 20% oxygen. β-Actin serves as protein loading control. Data shown are representative of experiments repeated at least three times with similar results. Values are shown as mean and s.e.m.;P-values are determined by Student'st-test. Figure 5: Respiration is inversely related to DNA damage response in genetically unmodified cancer cells and primary fibroblasts. ( a ) Respiration in HCT116 SCO2+/+ cells was inhibited by acutely targeting each of the three respiratory complexes with the indicated agents for 24 h (I=rotenone, 0.1 μM; III=antimycin A, 3 mM; IV=potassium cyanide, 0.1 mM). DNA damage responses under indicated ambient oxygen conditions were monitored by γ-H2AX western blotting. As negative control, note the lack of DNA damage response in non-respiring SCO2−/− cells. ( b ) SCO2+/+ cells maintained under indicated oxygen conditions were FACS sorted by mitochondrial membrane potential using potentiometric dye JC-1 and divided into a low (L), medium (M) or high (H) mitochondrial membrane potential sub-population ( ∼ 5 to 10% of the total population). The viability of all three fractions was greater than 96–99% by Trypan blue dye exclusion. ( c ) The stability of the mitochondrial membrane potential of postsorted cells was confirmed by FACS at the same setting. ( d ) Whole-cell oxygen consumption measurements in L, M and H mitochondrial membrane potential sub-populations (nmol per min per 10 6 cells) ( n =3). ( e ) Relative ROS levels in the respective fractions quantified by DCF FACS ( n =3). ( f ) Relative DNA damage response in the respective fractions determined by γ-H2AX western blotting. ( g ) DNA damage response of primary mouse embryo fibroblasts under the indicated ambient oxygen conditions, as well as after FACS sorting into L, M and H mitochondrial membrane potential sub-populations in 20% oxygen. β-Actin serves as protein loading control. Data shown are representative of experiments repeated at least three times with similar results. Values are shown as mean and s.e.m. ; P -values are determined by Student's t -test. Full size image A key process that contributes to the maintenance of mitochondrial membrane potential is active respiration. This principle has been applied to the sorting of cells into sub-populations with differences in oxygen consumption capacity by the use of potentiometric dyes [34] , [35] . We used the mitochondrial membrane potential indicator 5,5′,6,6′-tetrachloro-1,1′,3,3′-tetraethyl-imidacarbocyanine iodide (JC-1) to fractionate HCT116 cultures into sub-populations of low (L), medium (M) or high (H) membrane potential by fluorescence-activated cell sorting (FACS), thus sorting them by respiratory capacity ( Fig. 5b ). The stability of the mitochondrial membrane potential in these fractions after FACS sorting was confirmed by repeating the cytometric analysis of each sub-population using the same settings ( Fig. 5c ). Within these unmodified sub-populations of healthy growing cells, there was a striking inverse relationship between oxygen consumption and ROS levels ( Fig. 5d,e ). In parallel, the ROS levels corresponded well to γ-H2AX DNA damage response levels in 20% oxygen ( Fig. 5e,f ). Notably, the higher γ-H2AX levels observed in lower respiratory capacity cells were significantly attenuated by decreasing ambient oxygen (1.5 or 5% compared with 20%) ( Fig. 5f ), thereby reproducing the effects observed after stable genetic or acute chemical disruption of respiration. To demonstrate that our observations are also generalizable to non-transformed cells, we prepared mouse embryo fibroblasts and similarly fractionated these normally cycling cells by mitochondrial membrane potential. Again, we observed an inverse relationship between mitochondrial function and DNA damage response ( Fig. 5g ). In summary, we have used an isogenic pair of respiring and non-respiring human cell lines to establish the potential importance of mitochondrial respiration in preventing oxygen-associated DNA damage. Molecular oxygen serves as the essential substrate for ROS generation. By eliminating bioenergetic dependence on oxygen for growth, we have revealed its potential genotoxicity. The loss of respiration affects intracellular oxygen and redox homeostasis, thereby increasing ROS formation and oxidative DNA damage, a promoter of genetic instability that may help drive the multistep process of tumorigenesis. In this light, the previously reported positive regulation of respiration by p53 is conceptually concordant with its well-accepted role as guardian of the genome and with the previously described antioxidant functions of p53 [21] , [36] . We propose that oxygen consumption by respiration represents a fundamentally important function of the mitochondria, which is to guard against the genotoxicity of oxygen, independent of oxidative phosphorylation. Such a concept would be relevant to diverse biological processes including cell proliferation, differentiation, stem cell maintenance and senescence [7] , [37] , [38] , [39] . Genotoxic DNA damage can promote the outgrowth of cancer clones by promoting mutagenesis, but generally functions to suppress cell growth. This apparent paradox is the principle that underlies most conventional forms of cancer therapy. Oxygen levels could similarly cause a paradoxical effect on cell growth and tumorigenesis. Indeed, cancer cells engineered to overexpress myoglobin and therefore containing higher intracellular oxygen have been reported to exhibit suppressed growth when used to found xenograft tumours [40] . Although this observation may seem incongruent with our current model, tumorigenesis is a complex multistep phenomenon that likely involves varying requirements over a lifetime for cancer cell selection and survival. Thus, oxidative stress may have an important role by introducing genomic instability during tumour initiation; however, once a cancer cell is established, its ability to grow may be more dependent on survival- and growth-promoting factors such as HIF1-α, which is destabilized by oxygen [22] , [40] , [41] . The reduction of oxygen to water by mitochondrial respiration may represent the integration of two essential functions for aerobic life: coupling to oxidative phosphorylation for bioenergetic benefits and elimination of the essential ROS substrate for maintaining genomic stability. In this model, the overall level of oxidative stress would be determined by both the availability of oxygen under ambient conditions and its disposal. This study provides a rationale for future investigations into the genotoxic effects of oxygen and the development of strategies to reduce the deleterious effects of oxygen by improving mitochondrial function. Viable strategies for the prevention of cancer and other degenerative diseases could include decreasing oxygen exposure or increasing oxygen consumption by improving aerobic capacity. It is also tempting to speculate that enhanced genomic stability provided by increased mitochondrial respiration may contribute to the decreased incidence of lymphomas in mice overexpressing mitochondrial uncoupling proteins, and to the protective effect of aerobic exercise capacity with respect to not only cardiovascular diseases but also cancer [42] , [43] , [44] . Antibodies and reagents The monoclonal antibodies used were 8-oxoG (dilution ∼ 1:200, clone 483.15), phospho Ser-139 histone H2AX (γ-H2AX, dilution ∼ 1:2,000, clone JBW301) (Millipore); p53 (dilution ∼ 1:300, DO-1) (Santa Cruz Biotechnology); porin (VDAC, dilution ∼ 1:3,000) (Invitrogen); and β-actin (dilution ∼ 1:10,000, clone AC-15) (Sigma). The purified rabbit polyclonal antibodies used were: human COX10 (dilution ∼ 1:300) (Proteintech Group); and SCO2 (dilution ∼ 1:500) [17] . The following chemicals were obtained from Sigma: oligomycin, NAC, rotenone, antimycin A, potassium cyanide, 2-deoxy- D -glucose, JC-1 and tetramethylrhodamine methyl ester perchlorate. Cells and tissue culture Human colon cancer HCT116 and primary fibroblast WI-38 cell lines were obtained from ATCC. HCT116 cells were maintained using McCoy's 5A medium supplemented with 10% fetal bovine serum and penicillin/streptomycin (Invitrogen) in a 95% air/5% CO 2 tissue culture incubator unless indicated otherwise. The SCO2−/− cell line was created as previously described and maintained in 1.5% or indicated O 2 /5% CO 2 using a variable multigas incubator (Sanyo) [24] . Cell lines were allowed to attach for at least 24 h after plating before the initiation of experiments, and cell viability was determined by Trypan blue dye exclusion assay. Mouse embryonic fibroblasts were isolated from 13.5- to 14.5-day-old embryos as previously described [37] . Human osteosarcoma 143B ρ + and ρ o cells were kindly provided by Dr Eric A. Schon. Somatic cell homologous recombination The SCO2 gene was targeted by recombinant adeno-associated virus -mediated homologous recombination as previously described [24] . Briefly, SCO2+/− cells that are G418 resistant were transduced with recombinant adeno-associated virus containing a hygomycin-B resistance marker flanked by homology arms [17] , [24] . SCO2−/− clones were selected in either 1.5 or 20% oxygen and screened by genomic PCR. Lentivirus for gene knockdown and overexpression Nonspecific SCO2, or COX10 short hairpin RNA (OpenBiosystems) and SCO2 cDNA lentivirus were prepared (Sigma-Aldrich) [24] and used to transduce cells with puromycin (2 μg ml −1 ) selection for at least 14 days. Gene knockdown or overexpression was confirmed by western blot analysis. Metabolic measurements For oxygen consumption, cells were trypsinized and resuspended at 10×10 6 cells ml −1 in complete medium and measured in a 1 ml-volume stirred, sealed chamber using a Clark-type oxygen microelectrode at 37 °C [17] . For lactate production quantification, 10×10 6 trypsinized and cold PBS-washed cells were resuspended in 100 μl PBS containing 3 mg ml −1 glucose. Lactate production was measured at 37 °C for 0, 10, 20 and 30 min using the Lactate Reagent kit (Trinity Biotech PLC, Wickow, Ireland) [17] . ATP levels in SCO2+/+ or SCO2−/− cells grown for 3 or 6 days, respectively, in 12-well plates were measured using the ATP Determination Kit (Invitrogen). For oligomycin treatment, cells were plated at 10×10 4 per well of a 24-well plate in DMEM and allowed to attach overnight. Cells were washed with DMEM medium (without glucose) and oligomycin (10 μM) was added for 6 h as previously described [45] . For 2-deoxy- D -glucose sensitivity measurements, cells were grown in complete medium containing 1 mM pyruvate with increasing amounts of 2-deoxy- D -glucose for 4 days [46] . For measurement of respiration/glycolysis ratio, lentivirus-transduced and selected cells were plated overnight on XF24 cell culture microplates (Seahorse Bioscience) at 4×10 4 cells per well, and oxygen consumption rate (representing respiration) and extracellular acidification rate (representing glycolysis) were simultaneously measured for 3 min in XF assay media [47] . Cellular NADH measurements For relative quantification of intracellular NADH levels, cells were grown on 35 mm live-cell imaging dishes (Mattek). NADH ultraviolet fluorescence images were captured using a ultraviolet filter (375 nm) with ×40 objective lens on a Zeiss LSM 510 UV laser-scanning confocal microscope and analysed [48] . ROS measurements Cells were stained with 5 μM CM-H 2 DCFDA (Invitrogen) for 15 min at 37 °C, washed in PBS, trypsinized and resuspended at 1×10 6 ml −1 . DCF signal was observed and analysed by FACSCalibur and CELLQuest software (version 3.3, BD Biosciences). Cells were treated with 15 mM NAC for 24 h to examine its effect on ROS production. Cells were maintained for 7–10 days and DCF was stained in a 5% oxygen tissue culture incubator to determine the effect of reduced ambient oxygen on ROS levels. Flow cytometry After staining in JC-1 solution (2.5 μg ml −1 ) for 15 min at 37 °C, cells with the lowest (5%), middle (10%) and highest (5%) membrane potentials were collected using the MoFlo cell sorter and Summit software (Beckman Coulter). Postsorted mitochondrial membrane potential stability was confirmed using the same FACS settings. Potentiometric dye tetramethylrhodamine methyl ester perchlorate (25 nM) also confirmed a similar relationship between mitochondrial membrane potential and oxygen consumption result; these fractions were used for ROS measurements by DCF FACS to avoid wavelength overlap between DCF and JC-1. Intracellular oxygen measurement Intracellular oxygen concentrations were quantified using a recently developed water-soluble photostable metalloporphyrin-based oxygen probe (IC60N) coupled with fluorescence lifetime imaging microscopy [29] . Measurement is based on the ability of molecular oxygen to quench the excited state of the oxygen probe, with the degree of quenching being dependant on oxygen concentration. Cells were plated (2×10 4 cells ml −1 ) on 35 mm glass-bottomed live-cell imaging dishes (Mattek) for 24 h in complete McCoy's 5A medium. Before transfection, the medium was replaced with 1 ml of fresh medium to which 100 μl of 10 μM IC60N stock and 6 μl of Endo-Porter (Gene Tools, LLC) were added. Cells were incubated for 20 h and washed in phenol red-free medium. Fluorescence lifetime imaging microscopy was performed on subconfluent cultures, averaging lifetimes in 15 discrete regions per sample on an Axiovert 200 inverted fluorescence microscope with an LED module, modulated CCD camera (LaVision Biotech) and an oxygen-controlling apparatus (Pecon). Pulses (15×5,000 ms) from a 395 nm LED were used, followed by collection of emission after each pulse using a 630 nm long-pass filter at discrete delay times between 12 and 60 μs with a gate time of 20 μs. Delay times were calculated by single exponential fitting of a 15-point exponential decay of each pixel in a 1,024×1,024 pixel field. Calibration was carried out on the SCO2−/− cell line in atmospheric air ( ∼ 20.5%), with 5 and 0% oxygen. Both cell types were measured at 5% extracellular oxygen and treated with either 5 μM antimycin A or vehicle (0.125% DMSO final concentration in growth medium). Western blotting Protein samples were prepared by adding either RIPA buffer with protease inhibitor cocktail or SDS–PAGE protein sample buffer directly to cells and freezing on dry ice. Protein samples were heated for 5 min at 95 °C before resolving and western blotting. Primary antibodies were incubated overnight at 4 °C and horseradish peroxidase-conjugated secondary antibodies (dilution ∼ 1:10,000, Jackson Laboratory) were added at room temperature according to standard protocol. If applicable, quantifications were performed by densitometric scanning using ChemiDoc XRS and Quantity one software (version 4.6.2, Bio-Rad). Immunofluorescence staining Cells were allowed to attach for 24 h onto two-well chamber slides (Lab-Tek) at their optimal oxygen growth condition. After 48 h exposure to the indicated oxygen concentration, cells were washed with PBS, fixed in 2% paraformaldehyde PBS (Electron Microscopy Sciences), permeabilized in 0.2% Triton X-100 PBS and blocked with 5% serum (of secondary antibody species) at room temperature, incubated with an anti-8-oxoG antibody overnight at 4 °C and with Alexa Fluro594-labelled secondary antibody (Invitrogen) at room temperature. PBS washes (3×5 min each) were performed between all steps and images were captured using an Axioskop2 Plus fluorescence microscope with Axiovision software (version 4.6). Colony formation assay SCO2−/− cells were plated at indicated densities on six-well plates and cultured in a 1.5 or 20% oxygen tissue culture incubator. For NAC rescue of colony formation, SCO2−/− cells were incubated with 3 mM NAC in a 20% oxygen incubator. After 10–12 days, the plates were stained with crystal violet, and colonies were imaged and quantified. Statistical analysis P -values were calculated using Student's t -test and Fisher's exact test as indicated. How to cite this article: Hwang, P. M. et al . Mitochondrial respiration protects against oxygen-associated DNA damage. Nat. Commun. 1:5 doi: 10.1038/ncomms1003 (2010).